Histone acetylation controls the inactive X chromosome replication dynamics In mammals, dosage compensation between male and female cells is achieved by inactivating one female X chromosome (Xi). Late replication of Xi was proposed to be involved in the maintenance of its silenced state. Here, we show a highly synchronous replication of the Xi within 1 to 2 h during early-mid S-phase by following DNA replication in living mammalian cells with green fluorescent protein-tagged replication proteins. The Xi was replicated before or concomitant with perinuclear or perinucleolar facultative heterochromatin and before constitutive heterochromatin. Ectopic expression of the X-inactive-specific transcript ( Xist ) gene from an autosome imposed the same synchronous replication pattern. We used mutations and chemical inhibition affecting different epigenetic marks as well as inducible Xist expression and we demonstrate that histone hypoacetylation has a key role in controlling Xi replication. The epigenetically controlled, highly coordinated replication of the Xi is reminiscent of embryonic genome replication in flies and frogs before genome activation and might be a common feature of transcriptionally silent chromatin. Genome replication in higher eukaryotes is regulated both spatially and temporally, as clearly illustrated by the changing pattern of replication structures throughout S-phase [1] . Early in S-phase, the replication machinery is present as small foci well distributed within the nuclear interior. In the mid S-phase, the replication foci surround the nuclear and nucleolar peripheries. Finally, in the late S-phase, replication occurs within larger clusters at the nuclear interior and periphery [2] , [3] . Early-replicating chromatin largely coincides with the so called R-bands [4] and has been correlated with regions of high gene density [5] , high gene activity [6] and lower condensation levels [7] . In contrast, mid-replicating chromatin corresponds to G-bands, genomic regions with an overall lower gene density that contain facultative heterochromatic regions as well as tissue-specific genes. Finally, late-replicating regions correspond to C-bands, containing mainly (peri)centromeric heterochromatin regions, with a lower gene density and higher condensation levels. The distinct replication timing of different chromatin regions raises the question of how replication timing is controlled. Potential determinants of replication timing are the specific epigenetic properties that define the 'chromatin signature' of a given genomic region [8] . Important candidates, possibly acting in combinations, are histone modifications, histone variants, small nuclear RNAs, chromatin-associated proteins and DNA methylation. For instance, studies on monoallelically expressed genes have demonstrated that the transcriptionally active allele replicates earlier and exhibits increased histone H3/H4 acetylation as well as H3K4 methylation levels [9] . Moreover, in yeast, deletion of the histone deacetylase (HDAC) Rpd3 leads to increased acetylation levels at many origins of replication and subsequently to early initiation of replication [10] . Similarly, treatment of human cells with the HDAC inhibitor trichostatin A (TSA) results in earlier replication of imprinted genes [11] . To dissect the control mechanisms of the replication of diverse chromatin states, we chose the inactive X chromosome (Xi), the most prominent facultative heterochromatic region in mammals. Xi in female somatic cells is a well-known example for epigenetically silenced chromatin [12] . In embryonic stem (ES) cells, the X-inactive-specific transcript ( Xist ) gene is transcribed at low levels from both X chromosomes, whereas in somatic cells it is transcribed exclusively from the inactive homologue, where it coats the chromosome territory [13] , [14] . Xist RNA accumulation, shown to be dispensable for maintaining the inactive state [15] , is initially followed by trimethylation of lysine 27 on histone H3 (H3K27m3) [16] , [17] and later by histone hypoacetylation [18] , DNA methylation [19] and the formation of the Barr body [20] . These modifications form a multilayer silencing mechanism proposed to maintain the silenced state of Xi [21] . Interestingly, in early studies using modified nucleotides to label replicating DNA of human blood cells [22] , [23] , [24] and postimplantation mouse embryonic cells [25] , [26] , the replication timing of Xi has been shown to differ from that of its active homologue (Xa). Analysing chromosomes in subsequent mitosis revealed that one of the two X chromosomes in female cells replicated later than all other chromosomes [24] . The 'late replication' of Xi has since then been referred to many times, and is to date thought to be an important factor for the maintenance of the silenced state [27] . In this study, we assessed the dynamics of Xi replication in living cells. Furthermore, we elucidate the epigenetic factors that determine this replication mode. To address these questions, we utilized green fluorescent protein (GFP)-tagged DNA replication factors to analyse the precise progression of S-phase in vivo , with high temporal and spatial resolution. We found Xi to replicate within a limited time period during early–mid S-phase and corroborated these results using classical nucleotide incorporation detection. We were further able to show that an autosome silenced by ectopic Xist expression acquires the same replication mode as Xi. Finally, we demonstrate that the level of histone acetylation is the critical factor controlling the maintenance of the replication timing of Xi. We conclude that in female mammalian cells, the Xi replicates in a synchronous manner, before constitutive heterochromatin, and these replication dynamics are controlled by histone hypoacetylation. Xi replicates synchronously during early–mid S-phase To identify replicating X chromosomes in mouse C2C12 cells, we detected labelled nucleotides (BrdU) in combination with fluorescence in situ hybridization (FISH) using X-chromosome-specific probes. 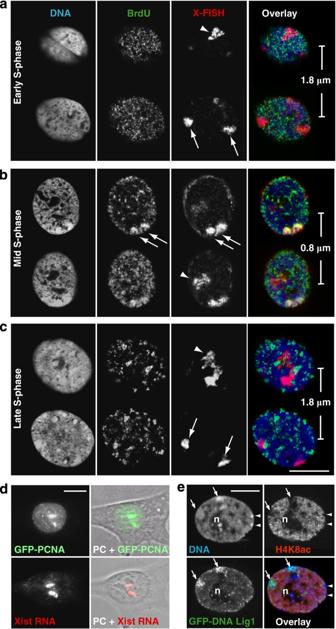Figure 1: Large mid S-phase replication structures represent bulk chromatin of the inactive X chromosome. C2C12 cells were BrdU pulse-labelled (10 μM, 30 min) to visualize actively replicating DNA, whereas the X chromosome was detected by FISH. DNA was counterstained using TO-PRO 3. Panels show two mid-confocal optical sections of three cells during (a) early, (b) mid or (c) late S-phase. Arrows point to the Xi territories. Arrowhead points to the Xa territory. Perpendicular scale bars indicate section distances in Z direction. (d) C2C12 cells expressing GFP-PCNA grown on photoetched coverslips featuring an alpha-numerical grid. Individual cells were pre-imaged for characteristic mid S-phase replication structures and postprocessed for FISH. After hybridization and detection of a Xist specific probe, cells were re-imaged to compare the localization of the GFP-PCNA and the Xist label. Xist and GFP-PCNA labelled the same chromatin regions within the nucleus. (e) Mid S-phase replication structures are hypoacetylated for histone H4 at lysine 8. Confocal microscopy images of a C2C12 cell stably expressing GFP-DNA ligase 1 show the characteristic large mid S-phase replication structures (arrows). The cell was stained with an antibody specific for H4K8ac. Note that the replication structures are clearly hypoacetylated, although the DNA staining by TO-PRO 3 indicates a dense, heterochromatic constitution, both hallmarks of the inactive X chromosome. Other heterochromatic regions show likewise reduced H4K8 acetylation levels (arrowheads). Scale bar, 10 μm. n: nucleolus; PC, phase contrast. Figure 1a–c depicts optical sections of mouse cells in early, mid and late S-phase. During mid S-phase, two X chromosomes colocalize with two large replication structures ( Fig. 1b , arrows), while the X chromosome in the lower optical plane ( Fig. 1b , arrowhead) shows very low replication labelling. In early and late S-phase cells, the two X chromosomes show essentially no overlap with replication sites ( Fig. 1a,c , arrowheads), whereas X chromosome material in Figure 1a,c (arrows) shows some degree of co-staining. We hypothesized that the two chromosome territories that colocalize with the prominent replication structures seen in mid S-phase ( Fig. 1b , arrows) could be the Xi differing in its replication timing from that of the active homologue. This hypothesis was supported by the fact that Xi stained by DNA dyes is highlighted as a densely labelled, compact structure, the so-called Barr body ( Fig. 1b,c , arrows); the putative Xi can be clearly characterized as Barr bodies. However, the appearance of two such structures can only be explained by a tetraploid karyotype, leading to the inactivation of two out of four X chromosomes [28] . A karyotype analysis of the transgenic C2C12 cell lines [29] indeed revealed an almost tetraploid chromosome composition, including four copies of the X chromosome ( Supplementary Fig. S1 ). Figure 1: Large mid S-phase replication structures represent bulk chromatin of the inactive X chromosome. C2C12 cells were BrdU pulse-labelled (10 μM, 30 min) to visualize actively replicating DNA, whereas the X chromosome was detected by FISH. DNA was counterstained using TO-PRO 3. Panels show two mid-confocal optical sections of three cells during ( a ) early, ( b ) mid or ( c ) late S-phase. Arrows point to the Xi territories. Arrowhead points to the Xa territory. Perpendicular scale bars indicate section distances in Z direction. ( d ) C2C12 cells expressing GFP-PCNA grown on photoetched coverslips featuring an alpha-numerical grid. Individual cells were pre-imaged for characteristic mid S-phase replication structures and postprocessed for FISH. After hybridization and detection of a Xist specific probe, cells were re-imaged to compare the localization of the GFP-PCNA and the Xist label. Xist and GFP-PCNA labelled the same chromatin regions within the nucleus. ( e ) Mid S-phase replication structures are hypoacetylated for histone H4 at lysine 8. Confocal microscopy images of a C2C12 cell stably expressing GFP-DNA ligase 1 show the characteristic large mid S-phase replication structures (arrows). The cell was stained with an antibody specific for H4K8ac. Note that the replication structures are clearly hypoacetylated, although the DNA staining by TO-PRO 3 indicates a dense, heterochromatic constitution, both hallmarks of the inactive X chromosome. Other heterochromatic regions show likewise reduced H4K8 acetylation levels (arrowheads). Scale bar, 10 μm. n: nucleolus; PC, phase contrast. Full size image To test whether the prominent replication structures coincided with the Xi, we performed Xist RNA FISH. To simultaneously visualize DNA replication sites, we used transgenic mouse C2C12 myoblasts expressing GFP-tagged proliferating cell nuclear antigen (PCNA) [1] . Figure 1d shows that GFP-PCNA and FISH stained the same regions, demonstrating that the prominent replication structures observed during mid S-phase are indeed the replicating Xi chromosomes. Moreover, Figure 1e shows that this structure is hypoacetylated, which is another hallmark of the Xi. We next analysed the replication dynamics of Xi in living cells. Following GFP-PCNA dynamics during S-phase progression (1 frame per 20 min; Supplementary Movies 1 , 2 , 3 , 4 ), we were able to visualize cells in the first half of S-phase with the same prominent replication structures as that observed in fixed cells ( Fig. 1b ). These structures persisted for 1 to 2 h ( Fig. 2a ) and coexisted with a replication pattern constituted by small replication foci at the nucle(ol)ar periphery, usually referred to as a mid S-phase replication pattern [30] . The pericentric heterochromatin region belonging to Xi was replicated later in S-phase, concomitant to the pericentric heterochromatin of the autosomes. We confirmed that the large structures visualized by GFP-tagged PCNA represented sites of actively replicating DNA by pulse-labelling nascent DNA in the transgenic C2C12 cells with BrdU ( Fig. 2b ). 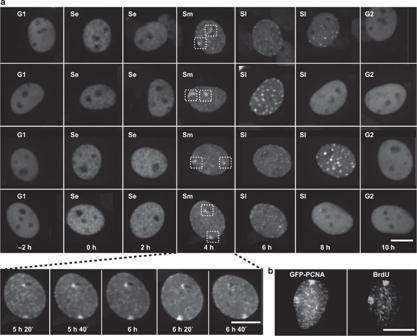Figure 2: The inactive X chromosome replicates synchronously during early–mid S-phase. (a) Selected frames of time-lapse imaging movies (Supplementary Movies 1,2,3,4) of C2C12 myoblasts stably expressing GFP-PCNA. Z-stacks were collected every 20 min over a time period of up to 15 h. GFP-PCNA1marks S-phase progression. Note the two large, synchronously replicating chromatin structures that appear during early–mid S-phase and persist for 60–120 min. (b) Epifluorescent micrographs of C2C12 cells stably expressing GFP-tagged PCNA. Cells were pulse-labelled with 10 μM BrdU for 30 min to visualize actively replicating DNA. Note that the large synchronously replicating DNA regions marked by PCNA were active sites of DNA synthesis as shown by the colocalization with incorporated nucleotide. Scale bar, 10 μm. Figure 2: The inactive X chromosome replicates synchronously during early–mid S-phase. ( a ) Selected frames of time-lapse imaging movies ( Supplementary Movies 1 , 2 , 3 , 4 ) of C2C12 myoblasts stably expressing GFP-PCNA. Z-stacks were collected every 20 min over a time period of up to 15 h. GFP-PCNA [1] marks S-phase progression. Note the two large, synchronously replicating chromatin structures that appear during early–mid S-phase and persist for 60–120 min. ( b ) Epifluorescent micrographs of C2C12 cells stably expressing GFP-tagged PCNA. Cells were pulse-labelled with 10 μM BrdU for 30 min to visualize actively replicating DNA. Note that the large synchronously replicating DNA regions marked by PCNA were active sites of DNA synthesis as shown by the colocalization with incorporated nucleotide. Scale bar, 10 μm. Full size image As BrdU incorporation alone provided a single time snapshot of the Xi replication, we performed a double nucleotide pulse, double chase experiment and let the cells enter into mitosis stage to analyse the distribution of the sequentially replicated regions in the mitotic chromosomes ( Fig. 3 ). Using X-chromosome-specific FISH (inset in Fig. 3 ), we were able to identify the sex chromosomes in the metaphase spreads and compare their replication in terms of the extent and distribution of replicated DNA. For this purpose, we applied a first pulse of 45 min with 5-iodo-2′-deoxyuridine (IdU; green signal in Fig. 3 ), followed by a 1 h 5-chloro-2′-deoxyuridine (CldU) pulse (red signal in Fig. 3 ) 2 h later and after 5.5 h, we prepared mitotic chromosomes. We observed two distinct populations of X chromosomes in each nucleus. Two X chromosomes (X 1 and X 1′ ) were labelled by both nucleotide pulses in a banded manner, similar to the autosomes, arguing for a discontinuous replication mode with only limited regions being replicated within a single-nucleotide pulse. The other two X chromosomes (X 2 and X 2′ ) showed only incorporation of the second label, with a higher proportion of chromatin being labelled compared with X 1 and X 1′ . The (peri)centromeric regions remained unlabelled, showing that the constitutive heterochromatic regions of these chromosomes are not replicated synchronously with the rest of the inactive territories. These findings offer a second independent line of evidence that the bulk chromatin of Xi (X 2 and X 2′ ) replicates in a synchronous mode within a limited time frame of about 1 h, whereas Xa (X 1 and X 1′ ) replicates similarly to the autosomes in a discontinuous manner throughout S-phase. Thus, we conclude that Xi in differentiated mouse female cells replicates synchronously and during the first half of S-phase. 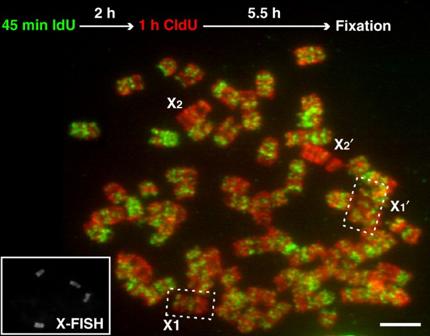Figure 3: Differential replication dynamics of Xa and Xi visualized in double replication labelled mitotic chromosomes. Mitotic spread of a C2C12 cell double labelled with IdU and CldU to simultaneously visualize DNA replicated at two time points with an interval of 2 h (see labelling scheme). X chromosomes were identified by FISH (see inset). Two X chromosomes show intense staining of most of their DNA, although having incorporated essentially only the second, that is, latter label (X2and X2′). The other two X chromosomes (X1and X1′) show a banded pattern of both labels, with only a limited incorporation of the later label. Scale bar, 10 μm. Figure 3: Differential replication dynamics of Xa and Xi visualized in double replication labelled mitotic chromosomes. Mitotic spread of a C2C12 cell double labelled with IdU and CldU to simultaneously visualize DNA replicated at two time points with an interval of 2 h (see labelling scheme). X chromosomes were identified by FISH (see inset). Two X chromosomes show intense staining of most of their DNA, although having incorporated essentially only the second, that is, latter label (X 2 and X 2′ ). The other two X chromosomes (X 1 and X 1′ ) show a banded pattern of both labels, with only a limited incorporation of the later label. Scale bar, 10 μm. Full size image Xi replication mode is conserved in mammals To test whether the Xi replication pattern we described above is a general feature of mammalian cells, we examined whether this replication pattern was also found in diploid primary cells, in cells of different tissues and in other species. Mouse primary cells were double labelled using a short 10 min pulses of IdU and CldU separated by a 3 h chase period ( Fig. 4a ), followed by a further 3 h chase period before they were fixed and immunostained for the incorporated IdU, CldU and DNA ligase 1, with the latter highlighting the state of DNA replication at the time of fixation [31] . Typically, cells that stained positively for all three replication markers displayed an early IdU, mid CldU and late DNA ligase 1 replication pattern and exhibited one prominent replication structure equivalent to that shown in Figures 1 and 2 , but only in the second, that is, mid-replication label and exclusively in female cells ( Fig. 4a ), confirming and extending our findings in mouse myoblasts. We co-stained sites of active replication and H3K27m3, a Xi hallmark, in mouse and human primary diploid fibroblasts to demonstrate that the prominent replication structure corresponds to the Xi ( Fig. 4b ). BrdU labelling of female diploid human vascular smooth muscle primary cells also revealed the presence of the large early–mid replication structure ( Fig. 4c ). On the basis of these observations, we conclude that the synchronous replication of Xi during the first half of S-phase is a phenomenon common to mammalian female cells and is not restricted to immortalized, aneuploid cell lines. 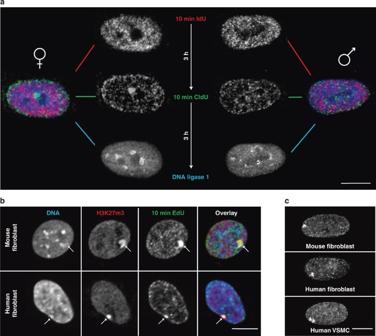Figure 4: Synchronous replication of Xi during early–mid S-phase is conserved in different types of cells and mammalian species. (a) Male and female primary mouse ear fibroblasts were triple-labelled to mark DNA replicated at three distinct time points during S-phase. The first two labels were accomplished by IdU and CldU incorporation, respectively, whereas the third time point was visualized by staining of DNA ligase 1. The chase time between the labels was 3 h. Shown are epifluorescent micrographs of a female and a male fibroblast exhibiting representative early (red), mid (green) and late (blue) replication pattern. (b) Co-staining of H3K27m3 and replication sites after 15 min of 10 μM 5-ethynyl-2′-deoxyuridine (EdU) incorporation in female primary mouse ear fibroblasts and human adult skin fibroblasts. (c) Xi replication pattern (see alsoa) in BrdU-labelled (100 μM, 20 min) female primary mouse ear fibroblasts, human fetal lung fibroblasts and human vascular smooth muscle cells (VSMC). Note that the characteristic Xi replication pattern coincides with the onset of the typical perinuclear mid S-phase replication pattern. Scale bar, 10 μm. Figure 4: Synchronous replication of Xi during early–mid S-phase is conserved in different types of cells and mammalian species. ( a ) Male and female primary mouse ear fibroblasts were triple-labelled to mark DNA replicated at three distinct time points during S-phase. The first two labels were accomplished by IdU and CldU incorporation, respectively, whereas the third time point was visualized by staining of DNA ligase 1. The chase time between the labels was 3 h. Shown are epifluorescent micrographs of a female and a male fibroblast exhibiting representative early (red), mid (green) and late (blue) replication pattern. ( b ) Co-staining of H3K27m3 and replication sites after 15 min of 10 μM 5-ethynyl-2′-deoxyuridine (EdU) incorporation in female primary mouse ear fibroblasts and human adult skin fibroblasts. ( c ) Xi replication pattern (see also a ) in BrdU-labelled (100 μM, 20 min) female primary mouse ear fibroblasts, human fetal lung fibroblasts and human vascular smooth muscle cells (VSMC). Note that the characteristic Xi replication pattern coincides with the onset of the typical perinuclear mid S-phase replication pattern. Scale bar, 10 μm. Full size image Xi replication timing is epigenetically controlled To examine the extent to which different epigenetic modifications define replication dynamics, we individually disrupted three epigenetic hallmarks of Xi: accumulation of Xist RNA, H3K27m3 and histone hypoacetylation. To assess the role of Xist expression in the synchronous Xi replication mode, we used mouse embryonic fibroblasts (MEF) carrying a Xist null allele on one homologue and a conditional knockout (KO; 'floxed') allele on the other chromosome (G19SV [15] , [32] ). This system allowed us to test whether accumulation of Xist RNA has an effect on the Xi replication dynamics. Using Cre recombinase-expressing adenoviruses (Adeno-Cre), we observed a complete loss of Xist expression in G19SV MEFs but not in control mock-infected cells, as shown by RNA FISH with a Xist-specific probe (data not shown). Loss of Xist expression had no influence on cellular proliferation ( Supplementary Fig. S2 ), in agreement with the published observations [15] , but resulted in a 50% reduction in the frequency of H3K27m3 Xi patterns ( Fig. 5a ), Moreover, knocking out Xist caused a significant increase in histone acetylation ( Fig. 5b ). Concomitantly, we observed a reduction in the percentage of Xi replication patterns (visualized by nucleotide incorporation) in Xist -deficient cells compared with control cells (4.7 versus 11.2%; Fig. 5c ). Xi replication mode was decreased by only 50% although Xist was absent in 100% of the cells, arguing against Xist being essential for the Xi replication dynamics and suggesting a connection between Xi replication pattern and downstream epigenetic modifications of the Xi. Indeed, in all Xist -deficient cells still displaying the typical Xi replication pattern, H3K27m3 still accumulated on Xi ( Supplementary Fig. S3 ). To assess the relationship between H3K27m3 and Xi replication dynamics, we used MEFs carrying two conditional KO alleles of the histone methyltransferase enhancer of zeste2 ( Ezh2 ; ref. 33 ) responsible for the H3K27m3 modification on Xi [16] , [17] . To induce recombination, the cells were incubated with the Adeno-Cre, followed by an additional growth period of 7 days. The frequency of H3K27m3 Xi patterns in virus-treated cells versus control-infected cells decreased from 81.4 to 12.4%, demonstrating successful recombination of the floxed Ezh2 gene. A significant decrease was also observed in the percentage of cells with the Xi replication pattern in virus-infected S-phase cells (0.7 versus 8.9% in control cells; Fig. 5c ), indicating that, independently of Xist expression, H3K27m3 accumulation has an influence on Xi replication. In contrast to loss of Xist expression, loss of Ezh2 had a dramatic effect on the proliferation of the cells, as revealed by the reduction of actively replicating cells from 45.7 to 6.7% ( Supplementary Fig. S2 ), suggesting that a decrease in H3K27m3 levels impedes normal cell-cycle progression. 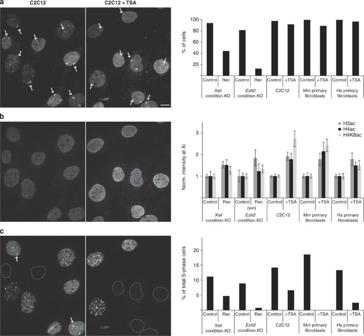Figure 5: Influence ofXist, H3K27m3 and histone acetylation on the Xi replication dynamics. Conditional KO MEFs forXist(G19SV) and for the histone methyltransferaseEzh2were used to determine the influence ofXistand H3K27m3 on the replication timing of Xi. The effect of hyperacetylation of Xi on its replication timing was analysed by treatment of C2C12 mouse myoblasts as well as mouse and human primary fibroblasts with 20 nM TSA over 4 days. Maximum intensity projections of control (left) and TSA-treated (right) C2C12 cells are presented to illustrate the quantification method. (a) Confocal images of cells immunostained with antibodies specific for H3K27m3. Arrows point to the cells scored as positive for H3K27m3 accumulation at Xi. Histogram shows the quantification of positive cells,n>220 for immortalized cell lines,n>34 for primary cells. (b) Confocal images of cells immunostained for H4K8ac. Histogram shows the intensity of Xi histone acetylation at H3ac, H4ac and H4K8ac, normalized to the respective control. In control and recombinedEzh2conditional KO cells, the whole nuclear (wn) histone acetylation was plotted. Error bars represent 95% confidence interval (c) Cells were labelled for 15 min with 10 μM EdU and incorporated nucleotide was detected. Arrows point to cells exhibiting the Xi replication pattern. Histogram shows the percentages of Xi replication pattern plotted relative to the total number of S-phase cells,n>85 for immortalized cell lines,n>20 for primary cells. Scale bar, 10 μm. Figure 5: Influence of Xist , H3K27m3 and histone acetylation on the Xi replication dynamics. Conditional KO MEFs for Xist (G19SV) and for the histone methyltransferase Ezh2 were used to determine the influence of Xist and H3K27m3 on the replication timing of Xi. The effect of hyperacetylation of Xi on its replication timing was analysed by treatment of C2C12 mouse myoblasts as well as mouse and human primary fibroblasts with 20 nM TSA over 4 days. Maximum intensity projections of control (left) and TSA-treated (right) C2C12 cells are presented to illustrate the quantification method. ( a ) Confocal images of cells immunostained with antibodies specific for H3K27m3. Arrows point to the cells scored as positive for H3K27m3 accumulation at Xi. Histogram shows the quantification of positive cells, n >220 for immortalized cell lines, n >34 for primary cells. ( b ) Confocal images of cells immunostained for H4K8ac. Histogram shows the intensity of Xi histone acetylation at H3ac, H4ac and H4K8ac, normalized to the respective control. In control and recombined Ezh2 conditional KO cells, the whole nuclear (wn) histone acetylation was plotted. Error bars represent 95% confidence interval ( c ) Cells were labelled for 15 min with 10 μM EdU and incorporated nucleotide was detected. Arrows point to cells exhibiting the Xi replication pattern. Histogram shows the percentages of Xi replication pattern plotted relative to the total number of S-phase cells, n >85 for immortalized cell lines, n >20 for primary cells. Scale bar, 10 μm. Full size image As loss of H3K27m3 resulted in an increase in histone acetylation, especially at histone H3 ( Fig. 5b ), we wondered whether H3K27m3 itself, being an early modification of Xi, is a direct determinant of the Xi replication dynamics or whether the possible concomitant loss of modifications downstream of H3K27m3, such as histone hypoacetylation, might be the actual cause for the decrease of Xi replication patterns in Ezh2 conditional KOs. To test this, we disrupted histone hypoacetylation [34] by treating cells with the HDAC inhibitor TSA, which leads to global histone hyperacetylation. As shown in Figure 5b , treatment with 20 nM TSA for 4 days, while not having a significant effect on the percentage of cells going through S-phase ( Supplementary Fig. S2 ), caused hyperacetylation of chromatin, both globally and directly at the Xi ( Supplementary Fig. S4 ). We found that the percentage of S-phase cells with the Xi replication pattern decreased from 13.3–18.6% in control cells to 0–6.6% in treated cells ( Fig. 5c ), suggesting that low acetylation levels on the Xi are required to maintain its synchronous early–mid replication timing. Importantly, TSA treatment did not cause the loss of H3K27m3 ( Fig. 5a ) or Xist RNA on Xi ( Supplementary Fig. S5 ), supporting a direct role of hypoacetylation in controlling Xi replication dynamics independently of Xist and H3K27m3. Thus, high H3K27m3 and histone hypoacetylation have a role in maintaining the characteristic synchronous early–mid replication timing of Xi, with histone hypoacetylation being the most likely to have a direct role. Inactive autosomes replicate as Xi upon cell differentiation As disrupting any of the Xi epigenetic modifications might have some influence on other epigenetic modifications [32] , we artificially controlled chromosome inactivation and followed the appearance of the distinct epigenetic modifications that accompany Xist -dependent whole-chromosome silencing. We monitored the relation of the epigenetic changes with the shift in the replication mode of the inactivated chromosome. We asked whether the ectopic expression of Xist from an autosome was sufficient to establish the characteristic synchronous, early–mid replication timing and whether we could temporally discriminate between the contribution of histone methylation and hypoacetylation to the inactive chromosome and their relation to synchronous replication. We used a male mouse transgenic ES cell line carrying a doxycycline-inducible Xist gene on chromosome 11. Previous studies have shown that Xist -expressing, silenced autosomes acquire a delayed replication timing only after cellular differentiation [35] . Thus, ES cells were induced to express Xist by adding doxycycline, and were either differentiated using retinoic acid or kept in an undifferentiated state ( Fig. 6a ). At 6 days after induction of Xist, cells were BrdU labelled to visualize the Xi replication pattern, and Xist RNA FISH was performed to label the silenced autosome ( Fig. 6b ). Whereas we observed the typical synchronous early–mid replication pattern shown for Xi (compare BrdU signal shown in Fig. 6b 'differentiated cell' with, for example, Fig. 1 ) in differentiated cells, we were unable to find such a replication structure in undifferentiated ES cells, though we did observe early–mid S-phase cells with the characteristic perinuclear and perinucleolar replication pattern ( Fig. 6b 'ES cell'). Therefore, we conclude that Xist expression from an autosome is sufficient to trigger all downstream mechanisms that are necessary to establish the synchronous early–mid replication pattern in differentiated cells. 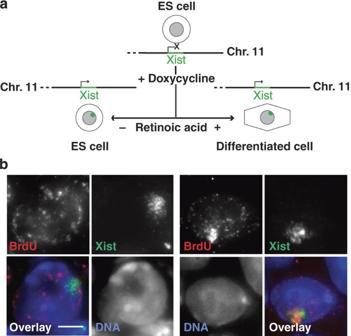Figure 6:Xist-dependent autosomal inactivation induces synchronous, early–mid replication in differentiated cells. (a) Mouse ES cells carrying an ectopic, doxycycline-inducibleXistgene on one chromosome 11 were either treated for 6 days with doxycycline and retinoic acid (differentiated,Xistexpressing) or singly with doxycycline (undifferentiated,Xistexpressing). (b) Cells were BrdU pulse labelled (10 min), fixed and stained to detect incorporated nucleotide followed by RNA FISH to detect Xist. DNA was counterstained with 4,6-diamidino-2-phenylindole. Epifluorescence micrographs show representative mid S-phaseXistexpressing ES (left) and differentiated (right) cells, as revealed by perinuclear BrdU specific staining. The characteristic Xi replication pattern was only observed in differentiated cells, but never in undifferentiated ES cells. Scale bar, 5 μm. Figure 6: Xist -dependent autosomal inactivation induces synchronous, early–mid replication in differentiated cells. ( a ) Mouse ES cells carrying an ectopic, doxycycline-inducible Xist gene on one chromosome 11 were either treated for 6 days with doxycycline and retinoic acid (differentiated, Xist expressing) or singly with doxycycline (undifferentiated, Xist expressing). ( b ) Cells were BrdU pulse labelled (10 min), fixed and stained to detect incorporated nucleotide followed by RNA FISH to detect Xist. DNA was counterstained with 4,6-diamidino-2-phenylindole. Epifluorescence micrographs show representative mid S-phase Xist expressing ES (left) and differentiated (right) cells, as revealed by perinuclear BrdU specific staining. The characteristic Xi replication pattern was only observed in differentiated cells, but never in undifferentiated ES cells. Scale bar, 5 μm. Full size image Histone acetylation regulates synchronous replication timing As cellular differentiation was required to establish the synchronous replication pattern of the inactivated autosome, we next examined the epigenetic differences before and after differentiation. Consistent with published data for Xi [16] , [17] and for the Xist -inactivated autosome [35] , [36] , accumulation of H3K27m3 was observed shortly after Xist induction ( Fig. 7a ) but before the appearance of the synchronous replication pattern. This result indicates that H3K27m3 is not sufficient to induce the shift in replication dynamics. Hence, we quantified the levels of histone acetylation at the inactivated autosome. We first selected the Xist -expressing autosome by the accumulation of H3K27m3 and analysed the histone acetylation level by plotting the variation of fluorescence intensity along a line across the inactivated chromosome territory ( Fig. 7b ). In addition, we performed a Pearson correlation analysis comparing the levels of H3, H4 and H4K8 acetylation at the inactivated autosome relative to the surrounding chromatin in ES versus differentiated cells. In all cases, this resulted in a significantly stronger anticorrelation in differentiated cells ( Table 1 ). Both analyses showed a clear decrease in histone acetylation level at the inactivated autosome upon differentiation, correlating with the appearance of synchronous replication patterns ( Fig. 7b ). Altogether, these observations (summarized in Fig. 7c ) confirmed our findings in somatic female cells and demonstrate that histone hypoacetylation directly promotes the rearrangement in replication dynamics of the inactive chromosome, whereas the Xist RNA coating and H3K27m3 per se are not sufficient to determine synchronous replication dynamics. 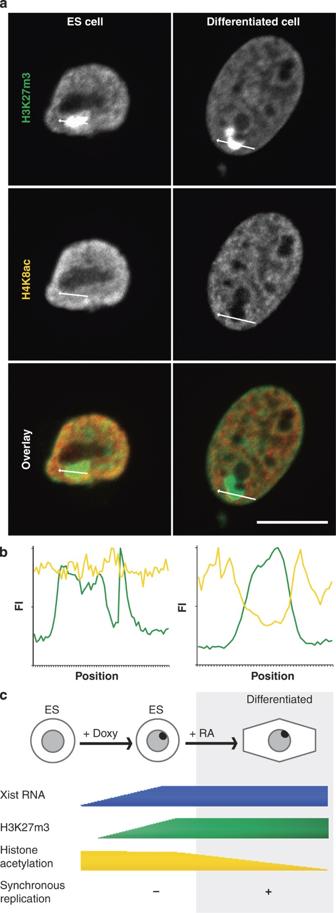Figure 7: Early–mid Xi replication pattern in differentiated cells correlates with global histone hypoacetylation on the inactivated autosome. (a) Undifferentiated ES or differentiated cells were fixed after induction ofXistand then double stained with antibodies to H3K27m3 and H4K8ac. Although accumulation of H3K27m3 at the inactivated autosome is already seen very clearly in undifferentiated cells (left), global histone hypoacetylation of this chromosome only appears upon differentiation (right). (b) Line intensity plots of H3K27m3 (green) and H4K8ac (orange) distribution through the inactivated autosome showing an increased anticorrelation of both epigenetic marks upon cellular differentiation. (c) Summary of the interplay between the different epigenetic modifications and their relationship to synchronous, early–mid replication before and after differentiation. FI: fluorescence intensity; RA, retinoic acid. Figure 7: Early–mid Xi replication pattern in differentiated cells correlates with global histone hypoacetylation on the inactivated autosome. ( a ) Undifferentiated ES or differentiated cells were fixed after induction of Xist and then double stained with antibodies to H3K27m3 and H4K8ac. Although accumulation of H3K27m3 at the inactivated autosome is already seen very clearly in undifferentiated cells (left), global histone hypoacetylation of this chromosome only appears upon differentiation (right). ( b ) Line intensity plots of H3K27m3 (green) and H4K8ac (orange) distribution through the inactivated autosome showing an increased anticorrelation of both epigenetic marks upon cellular differentiation. ( c ) Summary of the interplay between the different epigenetic modifications and their relationship to synchronous, early–mid replication before and after differentiation. FI: fluorescence intensity; RA, retinoic acid. Full size image Table 1 Pearson correlation coefficient for different acetylated residues in ES and differentiated cells. Full size table In the present study, we demonstrate that Xi in somatic mammalian cells replicates during early–mid S-phase. The replication of most of the silenced chromosome takes place in a synchronous manner, indicating the simultaneous firing of more replication origins than in the active homologue. Furthermore, we found that these replication dynamics are controlled epigenetically. Using a system [35] that permits temporal discrimination of the appearance of different modifications and their respective effect on the replication of the inactive chromosome, we found that an Xist -expressing autosome assumed the typical Xi-like synchronous replication only after cellular differentiation and global hypoacetylation of the silenced chromosome. Thus, we conclude that histone hypoacetylation is the most direct epigenetic determinant of the Xi replication mode. Our time-lapse analysis showed that the bulk of Xi replicates within a narrow time frame in early–mid S-phase. Earlier studies that defined Xi as late replicating [22] , [23] , [24] , [37] , [38] , [39] can be reconciled with our study by carefully considering the labelling protocols used. Using synchronized cultures, pulse labelled with tritiated thymidine shortly after the release of an S-phase block would exclusively label the early replicating DNA. In mitotic spreads of such pulse-labelled cultures, the lack of label on one of the X chromosomes was correctly interpreted as 'non-early' replication [38] , [39] . Increasing the nucleotide pulse duration to 3 h resulted in staining also the Xi [39] , which indicates that replication of the presumable Xi must have started 3 h after the release of the cell-cycle block. Schwemmle et al . [40] performed cell synchronization followed by (0.5–1 h) nucleotide pulse labelling and detected no nucleotide incorporation in the Xi during the first 1–2 h after release from G1/S block, and Xi replication was detected only thereafter. This study also reevaluates a series of reports, for example, refs 41 , 42 based on continuous labelling approaches describing a high variability in the replication sequence of the Xi. The authors could not corroborate the variation in the Xi replication sequence, which is likely a consequence of the variation in the length of the cell-cycle stages. Their results fit well with our time-lapse imaging and fixed cell data ( Fig. 2 and Supplementary Movies 1 , 2 , 3 , 4 ). Interestingly, replication studies performed in mouse embryonic cells at different days post coitum (d.p.c.) show a shift from isocyclic to allocyclic replication, with delayed initiation and early cessation of the Xi replication at 6.5 d.p.c. [25] , [26] . In a recent study, cells were double pulse labelled with a chase of 4 h in between and hybridized with an X-chromosome-specific paint [43] . Cells that incorporated modified nucleotides during both pulses were selected, with the first pulse labelling early and the second mid/late replication structures. In that report ( Fig. 2; ref. 43 ), the second pulse shows a typical mid pattern, including the synchronously replicating Xi, widely excluded from the first pulse. Our data do not exclude that small regions of the Xi might be replicated asynchronously from the Xi bulk chromatin, in agreement with the study by Hansen et al . [44] In contrast to autosomes and Xa, in which a limited number of origins fire at any given time during S-phase [45] , the number of firing origins engaged in replication of Xi appeared to be concentrated within a limited period of time ( Fig. 3 ). This previously suggested synchronous replication [24] is demonstrated both by our in vivo time-lapse analysis using fluorescently tagged replication factors as well as by nucleotide incorporation. As both X chromosomes contain the same DNA sequence and have been shown to utilize at least in part the same replication origins [46] , the synchronous replication dynamics cannot be explained genetically, suggesting that epigenetics have an important role in determining Xi replication dynamics. Indeed, we showed that the redundancy of Xist expression in the maintenance of transcriptional silencing [15] is paralleled by a partial redundancy in the maintenance of the Xi replication timing. Xist RNA accumulation is the first event during the initiation of X inactivation in differentiating cells [47] , hence knocking out Xist results in partial loss of downstream Xi modifications, such as H3K27m3 (refs 16 , 17 ), and consequently in partial loss of the synchronous replication pattern. Our observation that in Xist conditional KO cells H3K27m3 is lost following the loss of Xist expression to the same degree as the Xi replication pattern, as well as an increase in histone acetylation, indicates that the partial loss of synchronous replication was caused by an altered histone modification composition rather than by deficient Xist RNA accumulation itself. Moreover, cells with a 'normal' Xi replication pattern showed the 'normal' elevated H3K27m3 level on Xi, although we cannot rule out other potential indirect effects of the different epigenetic manipulations. Finally, we showed that the loss of histone hypoacetylation at Xi, as a consequence of HDAC inhibition by TSA, results in a significant decrease in synchronous replication, and that global histone hypoacetylation upon differentiation correlates with the appearance of the synchronous, early–mid Xi replication dynamics ( Fig. 7 ). Importantly, in TSA-treated cells, the levels of Xist RNA and H3K27m3 at the inactivated chromosome were normal and both modifications were also present in transgenic ES cells before differentiation and appearance of the synchronous replication pattern ( Fig. 7 ). Thus, Xist RNA and H3K27m3 are not sufficient to set the replication timing of the Xi and, hence, the most direct determinant of Xi replication dynamics is the level of histone acetylation. A possible consequence of the different timing of X chromosome replication, addressed in previous studies, could be that specific epigenetic marks on Xi have to be set within a limited window of time during early–mid S-phase, to limit the chromatin portion being modified [48] , with distinct histone modification outcomes depending on the replication timing and ultimately influencing and/or reinforcing the transcriptional state of the replicated chromatin. The immunodeficiency, centromere instability and facial anomalies (ICF) syndrome constitutes a striking example of the relationship between replication timing and transcriptional activity. In such cells, CpG islands of the Xi are hypomethylated [49] , but only those genes that replicate asynchronously from the bulk Xi and synchronously with the Xa homologue escape X inactivation [50] . The synchronous replication of Xi, implying the simultaneous firing of replication origins that in the active homologue fire sequentially [46] , resemble observations in embryos of flies and frogs previous to the onset of transcriptional activity. In Drosophila embryos, replication origins are regularly spaced and fire synchronously thus permitting entire genome duplication within the extraordinarily short (3–4-min-long) S-phase of the initial 10–13 mitotic divisions [51] . In Xenopus embryos, untranscribed DNA is replicated up to 11 times in only 7 h (ref. 52 ), requiring synchronous firing of all licensed replication origins and their regular distribution [53] , [54] to achieve an extremely fast completion of S-phase. Interestingly, this untranscribed chromatin is also hypoacetylated. One possibility could be that the absence of transcriptional activity/competence and the concomitant lack of necessity of coordinating both processes might allow simultaneous replication throughout transcriptionally silenced regions [55] . Altogether, we speculate that the synchronous replication dynamics of Xi might represent a common replication manner of different forms of transcriptionally silent chromatin and that histone hypoacetylation is the common epigenetic denominator regulating their replication synchrony. Cells C2C12 mouse myoblasts were grown at 37 °C/5% CO 2 in DMEM supplemented with 20% FCS and 1 μM ml −1 gentamycin [56] . A stable cell line expressing GFP-PCNAL2 [1] or GFP-DNA ligase 1 (ref. 31 ) was selected by a combination of fluorescence-activated cell sorting, antibiotic selection and screening for GFP-positive clones via fluorescence microscopy. Mouse primary fibroblasts were isolated from adult mouse (C57BL/6) ear tissue by cutting the ear tip with a scalpel. The tissue was shaken at 37 °C with 2 mg ml −1 collagenase NB8 (Serva Electrophoresis) in DMEM supplemented with antibiotics and vortexed repeatedly. Single cells were plated on a dish and cultivated in DMEM supplemented with 20% FCS at 37 °C/5% CO 2 . As human diploid female cells, we used fetal lung fibroblasts WI-38 (ref. 57 ) and fibroblasts established from a skin biopsy obtained from a young healthy female, kindly provided by the University of Amsterdam, as well as primary coronary artery smooth muscle cells (Cell System Biotechnologie Vertrieb GmbH; Cat.# CC-2583, Lot.# 15524). ES cells carrying a doxycycline-inducible Xist gene in chromosome 11 (ref. 35 ) were cultured, induced and either kept undifferentiated or differentiated for 6 days in the presence of 1,000 U ml −1 leukemia inhibitory factor (LIF) and feeder cells or 100 nM retinoic acid, respectively ( Figs 6 and 7 ). Xist expression was induced by 10 μg μl −1 . MEFs carrying two conditional KO ('floxed') alleles of Ezh2 were cultured and recombined using Adeno-Cre or Adeno-Cre-GFP (Vector Laboratories Inc.) virus as described [33] ( Fig. 5 ). Female SV40 T-antigen-transformed MEFs with a Xist deletion on one X chromosome and a 'floxed' allele on the other are described in ref. 32 and were cultured accordingly and recombined using Adeno-Cre virus as for Ezh2 MEFs ( Fig. 5 ). To induce histone hyperacetylation, C2C12 myoblasts, as well as mouse and human primary fibroblasts, were treated with TSA at a final concentration of 20 nM for 4 days ( Fig. 5 ). Immunofluorescence Cells were grown on glass coverslips, fixed in 4% paraformaldehyde (10 min at room temperature (RT)) and permeabilized for 20 min at RT in 0.5% triton/PBS. Immunofluorescence staining was performed in 4% BSA/PBS for 1 h at RT (primary antibodies) and for 45 min at RT (secondary antibodies). The following primary antibodies were used: anti-DNA ligase 1 antibody (1/100; ref. 31 ), anti-acetylated histone H3 (1/200, Upstate, Cat. no. 06-599), anti-acetylated histone H4 (1/200, Abcam, Cat. no. 06-866), anti-acetylated lysine 8 on histone H4 (1/500; ref. 18 , Upstate, Cat. no. 06-760) and anti-H3K27m3 (1/400, Upstate, Cat. no. 05-851). Nuclear DNA was visualized by Hoechst 33258 (1 μg ml −1 ), 4,6-diamidino-2-phenylindole (0.05 μg ml −1 , Sigma-Aldrich) or TO-PRO-3 (1 μM, Invitrogen). Cells were mounted in Vectashield antifade (Vector Laboratories Inc.). In situ replication labelling To visualize replicating DNA, cells were pulse labelled with 5-bromo-2′-deoxyuridine (Sigma-Aldrich) or 5-ethynyl-2′-deoxyuridine (Invitrogen), or double pulse labelled using 5-iodo-2′-deoxyuridine (20 μM IdU, 30 min, Sigma-Aldrich) and 20 μM CldU (30 min, Sigma-Aldrich) with a chase of 2–3 h after each pulse. For the preparation of double labelled mitotic chromosomes, replicating DNA of C2C12 cells was double labelled by applying a first 45 min IdU pulse followed by washing and incubation in conditioned medium for further 2 h before applying a second CldU pulse for 60 min ( Fig. 3 ). After washing extensively, cells were allowed to grow for an additional 5.5 h including colcemid treatment (30 min, 0.08 μg ml −1 ) before preparation of mitotic chromosomes according to standard procedures. Halogenated nucleotides were detected using anti-BrdU/IdU (1/100, clone B44; Becton Dickinson) and anti-BrdU/CldU (1/50, clone BU1/75, Serotec) antibodies or the ClickIT detection system as recommended by the manufacturer (Invitrogen). FISH Three-dimensional FISH ( Fig. 1a–c ) and metaphase FISH ( Fig. 3 ) with mouse chromosome paints [58] were performed according to standard protocol [59] . For three-dimensional FISH, cells were, in addition to the fixation steps described for immunostaining, incubated in 20% glycerol for 45 min, frozen and thawed in liquid N 2 four times, treated with 0.1 N HCl for 5 min and kept in 50% formamide/2× SSC overnight. For RNA FISH with Xist probes, 0.1 N HCl treatment was omitted ( Figs 1d and 6b and Supplementary Fig. S5 ). The probe for mouse Xist RNA detection was a PCR product of exon 1 and 6 from a cosmid-cloned Xist gene [60] . Full-length human Xist complementary DNA was purchased from Origene (cat. no. SC312039). Combination of FISH and halogenated nucleotide detection ( Figs 1 , 3 , 6 ) was performed by sequential detection of the modified nucleotides without additional denaturation after standard FISH detection. C2C12 cells expressing GFP-PCNA were subcultured on coverslips engraved with a photoetched alpha-numerical grid (Bellco) to identify and image the same cells in vivo (for GFP signal), and after FISH procedure to identify the inactive chromosome ( Fig. 1d ). Microscopy Epifluorescence images were obtained using Zeiss (Zeiss) Axiophot II and Axiovert 200 microscopes equipped with Zeiss Plan-Apochromat ×63/1.4 numerical aperture (NA) oil immersion objective lenses and CCD cameras. Confocal images were collected using an UltraVIEW VoX spinning disc system on a Nikon Ti microscope equipped with an oil immersion Plan-Apochromat ×60/1.45 NA objective lens (pixel size in XY=111 nm, Z-step=0.3–1 μm) or a Leica TCS SP1 or SP5 confocal laser scanning microscope (Leica) equipped with an oil immersion Plan-Apochromat ×63/1.4 NA objective lens (pixel size in XY set to 50 nm, Z-step=200 nm). Axial chromatic shift was corrected and corresponding RGB stacks, montages and maximum intensity projections were created using ImageJ ( http://rsb.info.nih.gov/ij/ ). Live-cell microscopy and mitotic shake-off Before live observation, cells were synchronized via mitotic shake-off ( Fig. 2 ). Growing medium was replaced by PBS/EDTA, and the adherent growing cells were shaken until most mitotic cells had detached from the substrate, as monitored on the microscope. The detached cells were re-plated on a microscopy dish and incubated under standard conditions for 5 h. G1 cells were then imaged. Four-dimensional time-lapse experiments were carried out on a UltraVIEW VoX spinning disc confocal system (PerkinElmer) in a closed live-cell microscopy chamber (ACU control, Olympus) heated to 37 °C, with 5% CO 2 and 60% air humidity control, mounted on a Nikon Ti microscope (Nikon). Image acquisition was performed using a ×60/1.45 NA Planapochromat oil immersion objective lens. Images were obtained with a cooled CCD camera. Maximum intensity projections were assembled onto QuickTime videos and annotated using ImageJ and Adobe Photoshop ( Supplemenatry Movies 1 , 2 , 3 , 4 ). Image analysis and quantification Quantification of the effects of drug treatment/virus infection/expression of Xist on replication mode ( Fig. 5 ) was assessed by comparing the frequency of the characteristic Xi replication pattern after BrdU incorporation. The levels of histone acetylation at the inactive territory were quantified by selecting the H3K27m3 accumulation as a region of interest (ROI) and measuring the mean intensity of the acetylation signal in the respective region. For Ezh2 conditional KO, the total nuclear histone acetylation signal was quantified, as the Xi lost its H3K27m3 accumulation. The (anti)correlation between histone acetylation and methylation signals at the inactivated autosome ( Fig. 7 ) was determined by plotting the normalized signal intensities at each pixel along a line through the inactive territory, as defined by accumulation of H3K27m3. The Pearson correlation coefficient was calculated using ImageJ within a region of interest containing the inactive chromosome and surrounding nucleoplasmic signal ( Table 1 ). How to cite this article: Casas-Delucchi, C. S. et al . Histone acetylation controls the inactive X chromosome replication dynamics. Nat. Commun. 2:222 doi: 10.1038/ncomms1218 (2011).